Functional ferroic heterostructures with tunable integral symmetry The relation between symmetry and functionality was pinpointed by Pierre Curie who stated that it is the symmetry breaking that creates physical properties. This fundamental principle is nowadays used for engineering heterostructures whose integral symmetry leads to exotic phenomena such as one-way transparency. For switching devices, however, such symmetry-related functionalities cannot be used because the symmetry in conventional heterostructures is immutable once the material has been synthesized. Here we demonstrate a concept for post-growth symmetry control in PbZr 0.2 Ti 0.8 O 3 and BiFeO 3 -based heterostructures. A conducting oxide is sandwiched between two ferroelectric layers, and inversion symmetry is reversibly switched on or off by layer-selective electric-field poling. The generalization of our approach to other materials and symmetries is discussed. We thus establish ferroic trilayer structures as device components with reversibly tunable symmetry and demonstrate their use as light emitters that can be activated and deactivated by applying moderate electric voltages. The correspondence of symmetry and functionality pervades all fields in physics and is a cornerstone for optimizing the performance of functional materials for technological applications [1] , [2] , [3] . Symmetry violations in time and space, for instance, are a hallmark for the emergence of magnetic and electric long-range order, respectively. If both of these symmetries are broken, novel interactions like magnetoelectric coupling effects are activated. A promising pathway towards enhanced or novel functionalities is to incorporate such symmetry violations directly into the material design. This is possible with high-end deposition techniques that allow for symmetry engineering at the atomic level by growing atomically sharp interfaces [3] , [4] . Growth-induced inversion symmetry violation, for example, can activate second-order nonlinear optical and first-order electro-optical phenomena, and broken time-reversale symmetry leads to Faraday and Kerr rotation [5] . A particularly elegant way for generating the desired symmetry reduction and inducing the aforementioned optical effects, or other unusual material properties, is acquired in so-called tricolour superlattices. In these tricolour superlattices, a geometric inversion symmetry breaking is achieved by the stacking of three constituents, A–B–C, as illustrated in Fig. 1a (refs 6 , 7 , 8 , 9 , 10 , 11 , 12 ). Unfortunately, a growth-based compositional symmetry breaking of the ABC-type is inevitably immutable: it cannot be altered after the completion of the growth process. In this sense, ABC-type heterostructures following the classical device paradigm may be regarded as passive building blocks. Here the step toward active heterostructures in which symmetry-driven functionalities can be repeatedly switched on and off via reversible post-growth symmetry control would be a major achievement. 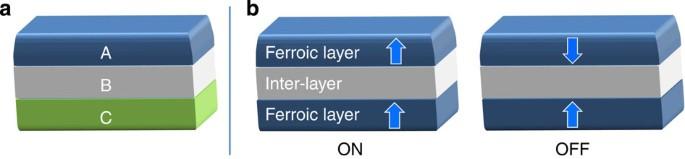Figure 1: Concept of reversible symmetry breaking in ferroic heterostructures. (a) Classical ABC-trilayer arrangement. (b) ABA trilayer for which the integral inversion symmetry is actively set to ON or OFF by parallel or antiparallel orientation of the ferroic order parameter. Figure 1: Concept of reversible symmetry breaking in ferroic heterostructures. ( a ) Classical ABC-trilayer arrangement. ( b ) ABA trilayer for which the integral inversion symmetry is actively set to ON or OFF by parallel or antiparallel orientation of the ferroic order parameter. Full size image In this article, we report such reversible post-growth symmetry control using epitaxial trilayer heterostructures with controllable inversion-symmetry properties as model system. We sandwich different oxide compounds between two ferroelectric layers and violate or retain the integral inversion symmetry of the trilayer system by controlling the associated polarization configuration as sketched in Fig. 1b . We demonstrate that such trilayer systems can act as nano-sized light emitters, which can be activated or deactivated at room temperature by applying moderate voltages rendering them promising candidates for electrically tunable sources in optoelectronic devices. Oxide trilayers with tunable integral symmetry For realizing symmetry-tunable heterostructures, we selected the textbook ferroelectric PbZr 0.2 Ti 0.8 O 3 (PZT) as constituent providing the symmetry environment and metallic La 0.7 Sr 0.3 MnO 3 (LSMO) as interlayer. Epitaxial PZT(001) (50 nm)/LSMO(001) (5 nm)/PZT(001) (50 nm) trilayers were grown on (001)-oriented SrTiO 3 (STO) substrates by pulsed laser deposition. The PZT thickness was set to 50 nm to retain the epitaxial strain imposed by the substrate and thus maintain a ferroelectric single-domain state [13] . 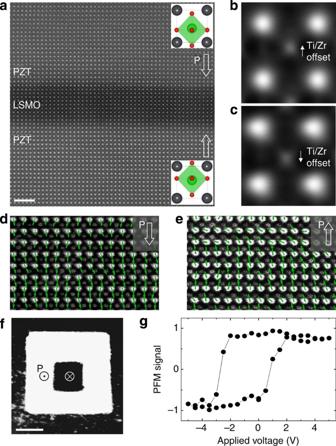Figure 2: Ferroelectric trilayer properties. (a) HAADF scanning transmission electron microscopy cross-section image (Z-contrast) of a PZT/LSMO/PZT trilayer (50/5/50 nm). Scale bar, 2 nm. Schematic insets inaillustrate the Zr/Ti cation displacements visible in the averaged structure images shown inbandc. White arrows indicate the direction of the associated spontaneous polarization. (d,e) Offset of the Pb and Zr/Ti sublattices with green arrows indicating the Pb displacement direction (see Methods). (f) Selective ferroelectric polarization switching in the upper PZT layer. Out-of-plane PFM image of an electrically switched box-in-box area. Scale bar, 1 μm. (g) Corresponding quasistatic normalized piezoresponse hysteresis loop. Figure 2a shows a cross-section of the PZT/LSMO/PZT trilayer system imaged by high-angle annular dark field (HAADF) scanning transmission electron microscopy. The image ( Z -contrast) reveals high-quality interfaces without any evidence of interdiffusion. Moreover, the direct visualization of the structure allows to determine the trilayer polarization state, which manifests as a cation (Ti/Zr) off-centring along the [001] growth direction in the PZT unit cells. This offset is visible in Fig. 2b,c , which show averaged structure images of the upper and lower PZT layer of Fig. 2a , respectively. A systematic analysis is provided in Fig. 2d,e presenting the local Pb-shift directions (green arrows) with respect to the Zr/Ti lattice as gained from fitting the atomic positions (see Methods). Based on Fig. 2b–e , we conclude that the polarization alternates according to + P ↔0↔− P across the LSMO interlayer with a sharp transition at the PZT/LSMO interfaces. Figure 2: Ferroelectric trilayer properties. ( a ) HAADF scanning transmission electron microscopy cross-section image ( Z -contrast) of a PZT/LSMO/PZT trilayer (50/5/50 nm). Scale bar, 2 nm. Schematic insets in a illustrate the Zr/Ti cation displacements visible in the averaged structure images shown in b and c . White arrows indicate the direction of the associated spontaneous polarization. ( d , e ) Offset of the Pb and Zr/Ti sublattices with green arrows indicating the Pb displacement direction (see Methods). ( f ) Selective ferroelectric polarization switching in the upper PZT layer. Out-of-plane PFM image of an electrically switched box-in-box area. Scale bar, 1 μm. ( g ) Corresponding quasistatic normalized piezoresponse hysteresis loop. Full size image Piezoresponse force microscopy (PFM) was applied to unveil the two trilayer polarization states in the PZT/LSMO/PZT system illustrated in Fig. 1b . We investigated the effect of applying an electric voltage of ±4 V to the top ferroelectric layer. Figure 2f shows the out-of-plane PFM contrast obtained after poling a box-in-box structure with the PFM tip. Bright and dark regions correspond to a ferroelectric single-domain state with + P and − P , respectively, clearly indicating that the upper layer can be selectively and reversibly switched between two stable ferroelectric states. This constitutes the two symmetry states illustrated in Fig. 1b . The locally acquired hysteresis loop in the piezoelectric (respectively ferroelectric) response shown in Fig. 2g reflects the excellent ferroelectric performance of the switchable PZT control layer. We note, however, that the negative bias of the local PFM loop in Fig. 2g indicates an influence on the PZT-switching behaviour exerted by the electrostatic environment or by interfacial strain [14] , [15] . This crosstalk suggests that the induced change of the integral symmetry may also be used to control the properties of the interlayer itself, for example, by activating spin-orbit coupling phenomena such as spin-band splitting (Rashba effect [16] , [17] , [18] ) or spin canting (Dzyaloshinskii–Moriya interaction [19] . ). In the following, however, we will focus on optical functionalities, considering the trilayer as an effectively homogeneous artificial material with tunable integral symmetry. Control of nonlinear optical activity An optical effect that directly relates to broken inversion symmetry is optical frequency doubling—also known as second harmonic generation (SHG). In the leading electric-dipole order, SHG can only occur when the integral trilayer inversion symmetry is broken [20] , [21] . This is described by the relation with the electric field E ( ω ) of the incident light wave at frequency ω , the induced electric-dipole oscillation P (2 ω) at frequency 2 ω , and the effective nonlinear susceptibility tensor of the trilayer system. For an antiparallel orientation of the polarization in the two PZT layers (OFF state in Fig. 1b ), the integral inversion symmetry is not violated so that . In contrast, the integral inversion symmetry is broken for parallel orientation of the polarization in the two PZT layers so that SHG is symmetry-allowed in this ON state ( ). In Fig. 3a , we present the optical response of an epitaxial PZT/LSMO/PZT trilayer grown on a SRO-buffered STO substrate at 620 nm when illuminated with light of 1240, nm wavelength. The spatially resolved data were taken after electrically poling an area of 80 × 80 μm 2 with a PFM tip. The poled area (dark) shows a distinct contrast level and is clearly distinguished from the surrounding region (bright). The cancelation of nonlinear optical activity in the poled area strikingly demonstrates that the electrically induced polarization reversal in the top PZT layer can be used to switch from a non-centrosymmetric (white↔ON) to a centrosymmetric (black↔OFF) state and hence control the optical trilayer properties. This switching behaviour further confirms that the top and bottom layers are decoupled, which is essential for manipulating the integral symmetry. In the present case, the decoupling is supported by conduction in the LSMO interlayer. The interlayer, however, does not have to be conducting: the decoupling of the control layers may as well be acquired via bias effects as seen in Fig. 2b or by pinning the polarization of the lower control layer, for example, by doping or an additional bottom electrode. 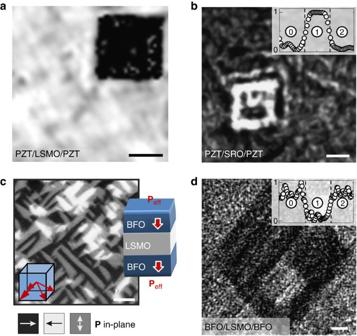Figure 3: Reversible control of the integral symmetry in ferroic oxide heterostructures. (a) Spatially resolved SHG data taken on PZT/LSMO/PZT after electrically poling a box with a PFM tip. Scale bar, 50 μm. (b) SHG image of an electrically poled box-in-box taken on PZT/SRO/PZT. Scale bar, 20 μm. As shown in the inset, the SHG yield (vertical axis) can be reversibly switched between two discrete levels. Numbers indicate the state at the start of the experiment 0, as well as the states obtained after the first 1 and second 2 polarization reversal. (c) In-plane PFM image of a BFO/LSMO/BFO trilayer system revealing four characteristic domain variants in the upper BFO layer. Schematic illustrations show the corresponding polarization directions (red arrows) and BFO/LSMO/BFO trilayer state. Scale bar, 500 nm. (d) Corresponding spatially resolved SHG data imaged after poling a box-in-box. Scale bar, 10 μm. The reversibility of the switch is depicted in the inset showing the SHG yield obtained in states 0, 1 and 2. Figure 3: Reversible control of the integral symmetry in ferroic oxide heterostructures. ( a ) Spatially resolved SHG data taken on PZT/LSMO/PZT after electrically poling a box with a PFM tip. Scale bar, 50 μm. ( b ) SHG image of an electrically poled box-in-box taken on PZT/SRO/PZT. Scale bar, 20 μm. As shown in the inset, the SHG yield (vertical axis) can be reversibly switched between two discrete levels. Numbers indicate the state at the start of the experiment 0, as well as the states obtained after the first 1 and second 2 polarization reversal. ( c ) In-plane PFM image of a BFO/LSMO/BFO trilayer system revealing four characteristic domain variants in the upper BFO layer. Schematic illustrations show the corresponding polarization directions (red arrows) and BFO/LSMO/BFO trilayer state. Scale bar, 500 nm. ( d ) Corresponding spatially resolved SHG data imaged after poling a box-in-box. Scale bar, 10 μm. The reversibility of the switch is depicted in the inset showing the SHG yield obtained in states 0, 1 and 2. Full size image Note that the concept for active inversion symmetry control and the aforementioned activation and deactivation of light emission by ferroelectric poling is not restricted to the case of PZT/LSMO/PZT trilayers. As suggested by Fig. 1b , it is a universal approach in the sense that no restrictions apply regarding the materials that are chosen as the interlayer and ferroelectric control layers. To verify the general validity, we realized different trilayer compositions by exchanging, in two separate variations, either the material used for the interlayer or the ferroelectric control layers. We begin with a discussion of the effects observed when replacing LSMO for SRO. The PFM analysis on pulsed laser deposition-grown high-quality PZT/SRO/PZT trilayers on STO (001) revealed that the top PZT layer grows in a ferroelectric mono-domain state and can be reversibly switched by applying a voltage of ±4 V to the PFM tip (not shown). In Fig. 3b , we present the nonlinear optical response measured on a PZT/SRO/PZT trilayer (50/25/50 nm) after electrically poling a box-in-box structure. Light emission (620 nm) from poled and unpoled areas is clearly different and, analogous to the case of LSMO, relates to the local symmetry state of the system (dark↔centrosymmetric, bright↔non-centrosymmetric). This evidences that the substitution of the interlayer material has no fundamental influence on the basic trilayer performance of Fig. 1b , so that we have the freedom to choose the interlayer material according to the desired functionality. In the next step, we replaced the ferroelectric PZT control layers by multiferroic BiFeO 3 (BFO) films while keeping the initial LSMO interlayer. In BFO, the coexistence of electric and magnetic order simultaneously violates space- and time-reversal symmetry. Thus, the use of BFO as control layer constituent allows, for example, to exploit the electronic and the spin degrees of freedom for tuning the trilayer symmetry. BFO/LSMO/BFO trilayers were grown on (001)-oriented STO substrates leading to four ferroelectric (multiferroic) in-plane variants with P ||〈111〉 resulting from the cubic symmetry of the substrate [14] , [22] . The four variants are visible in Fig. 3c showing a PFM scan of the BFO/LSMO/BFO trilayer. The associated domains, however, possess a lateral size in the order of 10–100 nm. As a consequence, the optical trilayer response is only determined by the effective out-of-plane polarization component, P eff , as sketched in Fig. 3c . From previous work, it is further known that P eff is accompanied by a collinearly oriented spontaneous magnetization [23] . M eff , which results from a canting in the antiferromagnetically arranged spins of the BFO films [24] . Thus, any reversal of P eff coincides with a reorientation of M eff which extends the symmetry control in our trilayers towards time reversal and the spin system. Regarding P eff , PFM scans performed on a BFO/LSMO/BFO trilayer (50 nm/30 nm/50 nm) revealed a homogeneous out-of-plane contrast for the upper BFO control layer. Figure 3d presents the corresponding nonlinear optical response detected after electrically poling a box-in-box structure with a PFM tip (±10 V). Similar to Fig. 3a , a striking decrease in light emission (620 nm) is observed when switching P eff (↔ M eff ) in the upper BFO control layer. It shows that the poling process reverses the integral space- and time-reversal symmetry state of the BFO/LSMO/BFO system. As a consequence, frequency doubling is deactivated in the poled area. A second electrical switch (inner box) then reactivates frequency doubling and leads to full recovery of the initial signal strength, which demonstrates that the symmetry violations in space and time are fully reversible. Integral symmetry of a trilayer assembly To consolidate that activated and deactivated emission of frequency-doubled light in our trilayer systems indeed relates to the integral symmetry expressed by , we also measured a model system that allows us to approach the geometry and symmetry of a complete trilayer system step by step. At first, PZT single layers with a thickness of 50 nm were grown on SrRuO 3 (SRO) buffered (001)-oriented STO. As indicated by the PFM image in Fig. 4a , the PZT grows in a ferroelectric single-domain state and can be reversibly switched by applying ±4 V to the PFM tip. In Fig. 4c–f , we show the corresponding SHG analysis performed with a standard transmission setup described elsewhere [20] . Analogous to the trilayer experiments, light at a photon energy around 1240, nm was incident at an angle of about 20° with respect to the surface normal of the PZT film. Because of the tilt, SHG components sensitive to the ferroelectric polarization along the [001] direction can be excited. A spatially resolved SHG measurement taken with SHG light from one of these components is presented in Fig. 4c . The black lines in the image retrace the ferroelectric 180° domain walls of the electrically poled box-in-box structure. This is further highlighted in Fig. 4b,d , which show the variation of the PFM and SHG contrast along cross-sections of the corresponding images. For modelling the lateral dependence I ( x ) of the SHG intensity, we calculated the local interference of SHG contributions from neighbouring domains with the spontaneous polarization + P and − P . Because of the linear coupling of the SHG susceptibility to the spontaneous polarization, the sign reversal of P is converted into a 180°-phase difference between SHG waves emitted from opposite domains [25] . 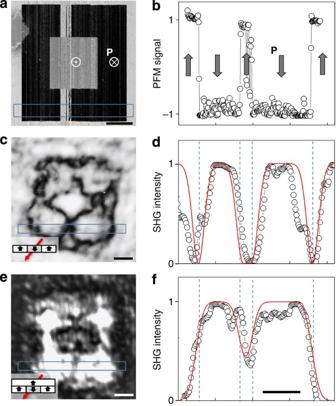Figure 4: Nonlinear optical response of a model trilayer. (a) Out-of-plane PFM image of an electrically switched area in a PZT/SRO heterostructure. Scale bar, 10 μm. (b) Normalized line scan of the section marked ina. (c) SHG image of the of poled area shown ina. Scale bar, 10 μm. A schematic of the ferroelectric domain pattern is shown as inset with the red arrow indicating the direction of the incident light beam. (d) Normalized line scan (black open dots) of the section marked incand calculated SHG intensity (red line). (e,f) Corresponding SHG image, normalized line scan and calculation for the model trilayer system sketched in the inset (see text for details). Scale bar, 10 μm. a.u., atomic unit. Thus, the net SHG yield for P =(0,0, P ) is given by Figure 4: Nonlinear optical response of a model trilayer. ( a ) Out-of-plane PFM image of an electrically switched area in a PZT/SRO heterostructure. Scale bar, 10 μm. ( b ) Normalized line scan of the section marked in a . ( c ) SHG image of the of poled area shown in a . Scale bar, 10 μm. A schematic of the ferroelectric domain pattern is shown as inset with the red arrow indicating the direction of the incident light beam. ( d ) Normalized line scan (black open dots) of the section marked in c and calculated SHG intensity (red line). ( e , f ) Corresponding SHG image, normalized line scan and calculation for the model trilayer system sketched in the inset (see text for details). Scale bar, 10 μm. a.u., atomic unit. Full size image Here sgn( P ( x ′)) accounts for the domain distribution in Fig. 4a and l =2.5 μm is entered as optical resolution. The good agreement between the SHG data and the calculated intensity profile in Fig. 4d corroborates that the SHG process is sensitive to the polarization state of the single 50-nm PZT layer investigated here. Taking advantage of this sensitivity, we then investigated the nonlinear optical response of an assembly that emulates the trilayer systems discussed earlier. A model trilayer was built by mounting the switched PZT film of Fig. 4a on top of a single-domain PZT/SRO/STO heterostructure with the two PZT layers facing each other. Measuring the nonlinear optical response on this model trilayer, we now obtained a pronounced difference in light emission at 2 ω leading to the contrast in the image shown in Fig. 4e . Because of the well-defined polarization state of the model trilayer (see inset to Fig. 4e ), the brightness levels can be unambiguously assigned to the local symmetry state. We find that dark regions correspond to a trilayer state with integral inversion symmetry, whereas bright regions are observed when the integral inversion symmetry is broken [26] . The good agreement between the SHG data and the calculated intensity profile in Fig. 4f confirms that the nonlinear optical response is determined by the ferroelectric polarization state in both the buried layer and the top layer. We demonstrated a concept for post-growth symmetry control in oxide materials using a trilayer geometry with adjustable ferroic control layers. As a model case, we discussed the activation and deactivation of light emission (optical frequency doubling) that was achieved by selective voltage-driven switching in one out of two ferroelectric control layers. Subsequent experiments demonstrated the generality of the approach. It is robust against an exchange of the control layers as well as the interlayer. By involving multiferroic BFO, we showed that even the type of environmental control is selectable. Aside from the integral spatial inversion exemplarily discussed in this work, it may involve the combined space and time reversal via multiferroic control layers (extending the classical spin-valve geometry [27] ) or strain tuning via ferroelastic control layers. The trilayer geometry may even be exploited to alter the local symmetry within the interlayer or at its interfaces. Our concept thus reveals a universal route for gaining control of electric, magnetic, distortive or even orbital degrees of freedom post growth. With this we create the basis for applications employing heterostructures as active device components, in which tailored functionalities driven by the integral symmetry can be switched on and off at will. Transmission electron microscopy The samples for our transmission electron microscopy measurements were prepared by mechanical wedge polishing and finally thinned by Argon ion milling using a Gatan PIPS. Scanning transmission electron microscopy was performed at the National Center for Electron Microscopy at Lawrence Berkeley National Lab on the TEAM0.5, an FEI titan G3 using a Cs probe corrector. Images were collected via a High-Angle Annular Dark Field Detector (HAADF). The PZT polarization direction was determined by the offset of the Pb and Zr/Ti sublattices using atomic positions extracted from a Gaussian fit to the HAADF data. Each data point is calculated as the offset vector between the central Pb atom and the mean position of the four surrounding neighbour Zr/Ti cations. Optical SHG SHG experiments were performed using 130 fs pulses of 1240, nm emitted at 1 kHz by an optical parametric amplifier pumped by a Ti:sapphire laser system. Pulse energies of about 5 μJ, that is, far below the sample’s damage threshold, were used and samples were investigated in a transmission setup using a LN 2 -cooled charge-coupled device camera. Leading-order SHG is parameterized by the nonlinear susceptibility tensors χ ijk ( P i (2 ω )= ε 0 χ ijk E j ( ω ) E k ( ω )) with i as polarization of the detected frequency-doubled light, and j and k for the incident light waves E ( ω ). The spontaneous polarization P =(0,0, P ) in the PZT films ( P || z ) allows for non-zero components χ zzz , χ zxx , χ zyy , χ xzx , χ yzy . For exciting these components, light was irradiated at a tilt angle α of about 20° with respect to the surface normal of the films. In trigonal BFO, additional crystallographic SHG components are symmetry-allowed due to the lower point-group symmetry (3m). The amplitude of the crystallographic background signal, however, is significantly smaller compared with the P -induced contributions when measuring a tilted sample ( α ≈20°) and can hence be neglected. How to cite this article : Becher, C. et al . Functional ferroic heterostructures with tunable integral symmetry. Nat. Commun. 5:4295 doi: 10.1038/ncomms5295 (2014).